One-dimensional surface phonon polaritons in boron nitride nanotubes Surface polaritons, which are electromagnetic waves coupled to material charge oscillations, have enabled applications in concentrating, guiding and harvesting optical energy below the diffraction limit. Surface plasmon polaritons involve oscillations of electrons and are accessible in noble metals at visible and near-infrared wavelengths, whereas surface phonon polaritons (SPhPs) rely on phonon resonances in polar materials, and are active in the mid-infrared. Noble metal surface plasmon polaritons have limited applications in the mid-infrared. SPhPs at flat interfaces normally possess long polariton wavelengths and provide modest field confinement/enhancement. Here we demonstrate propagating SPhPs in a one-dimensional material consisting of a boron nitride nanotube at mid-infrared wavelengths. The observed SPhP exhibits high field confinement and enhancement, and a very high effective index ( n eff ~70). We show that the modal and propagation length characteristics of the SPhPs may be controlled through the nanotube size and the supporting substrates, enabling mid-infrared applications. Surface phonon polaritons (SPhPs), the infrared (IR) counterparts to surface plasmon polaritons (SPPs), originate from coupling between electromagnetic waves and optical phonons of polar materials [1] , [2] , [3] , [4] . SPhPs and SPPs share similar traits: propagation along a boundary, high field density at the surface, a reduction of the guided wavelength (compared with free space) and spatial coherence of charge oscillations [5] , [6] , [7] , [8] , [9] , [10] , [11] , [12] . Noble metals have been widely used to support SPPs in the visible frequencies. However, in the mid-IR, noble metal SPPs evolve into Zenneck waves and their dispersion curves almost coincide with the light line. In general, the mid-IR spectrum is not easily accessible to metallic plasmonics [4] , [13] , [14] . Specially-designed structured surfaces and wires have been proposed to extend the surface plasmon into the mid-IR range; however, at a high fabrication complexity and cost [15] , [16] . Thus, SPhPs are highly desirable for extending nanophotonics into the mid-IR range. The creation of a surface polariton requires a negative real part in a material’s complex dielectric function [1] , [17] . Hexagonal boron nitride ( h -BN) has a strong phonon resonance that results in a negative permittivity band on the high frequency side of the resonance [18] , and has recently been found to be capable of supporting mid-IR SPhPs [19] . The multiwall boron nitride nanotubes (BNNTs) [20] , [21] , [22] , are a one-dimensional (1D) version of boron nitride, with geometry that can be controlled through chemical synthesis. BNNTs are chemically inert and mechanically strong with diameters as small as 2 nm. These chemical and morphological properties are not typically available to noble metals used in visible plasmonics, or other phonon polariton supporting polar materials such as SiC (ref. 23 ) or SiO 2 . BN in the form of nanotubes would provide a suitable geometry to confine and deliver IR energy in the form of SPhPs to a desired location at the nanoscale. Here, we report experimental observations and numerical simulations of 1D SPhP in BNNTs. The SPhPs in BNNTs are found to possess very high effective indices, surpassing that of SPPs in noble metals, and SPhPs in planar materials. The propagation characteristics of 1D SPhPs are found to be dependent on the geometry of the BNNTs, as well as the choice and structures of the supporting substrates. In particular, mitigation of SPhP loss can be achieved by using a rough metal substrate. The findings show the potential of BNNTs for utilizing 1D SPhPs. Observation of SPhPs in a BNNT Before experimental investigation, we carried out model calculations to estimate the possible performance of BNs as SPhP supporting materials. The dielectric function of h -BN is shown ( Fig. 1a ), calculated from the literature [18] . 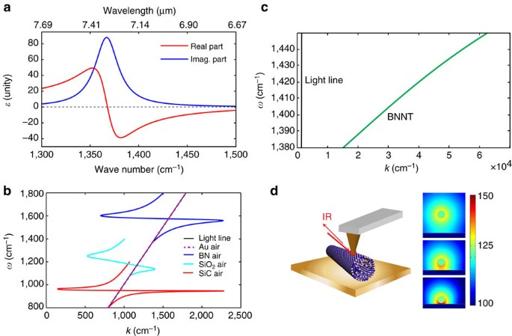Figure 1: Dielectric function of BN and s-SNOM. (a) Dielectric function of hexagonal BN. Strong phonon resonance leads to a negative region of the real part of the dielectric function. (b) Dispersion curves of SPhPs for flat interfaces of SiC, SiO2, BN and Au with air. (c) The dispersion curve of a 25-nmdiameter 1/3 hollow BNNT in air. (SeeSupplementary Note 1andSupplementary Fig. 1for a comparison of propagation lengths.) (d) Scheme of a near-field IR scattering with a metallic tip. The right-hand panels shows the spatial distribution of |E|, in dB, for the BNNT of partaat a distance of, respectively, 50, 10 and 3 nm above an Au plane, for a mode power normalized to 1 μW. The mode is highly confined between the BNNT and Au plane at a close distance. Figure 1b depicts the computed dispersion curves of SPhPs at a flat interface of SiC, SiO 2 , BN, and Au with air. All of these reside close to the light line, thereby offering long polariton wavelengths and modest confinement. Figure 1c presents the dispersion curve of a 25-nm diameter BNNT in air, whose SPhP wavenumber ( k ) is about an order of magnitude larger than those of the flat interfaces. These large wavenumbers indicate dramatic reduction of the guided wavelength, highly confined modes and considerable field enhancement for the 1D SPhP of a BNNT compared to SPhP in h -BN and other planar SPhP materials. The nanotube geometry leads to higher field confinement than that from the planar geometry. Figure 1: Dielectric function of BN and s-SNOM. ( a ) Dielectric function of hexagonal BN. Strong phonon resonance leads to a negative region of the real part of the dielectric function. ( b ) Dispersion curves of SPhPs for flat interfaces of SiC, SiO 2 , BN and Au with air. ( c ) The dispersion curve of a 25-nmdiameter 1/3 hollow BNNT in air. (See Supplementary Note 1 and Supplementary Fig. 1 for a comparison of propagation lengths.) ( d ) Scheme of a near-field IR scattering with a metallic tip. The right-hand panels shows the spatial distribution of |E|, in dB, for the BNNT of part a at a distance of, respectively, 50, 10 and 3 nm above an Au plane, for a mode power normalized to 1 μW. The mode is highly confined between the BNNT and Au plane at a close distance. Full size image Experimentally, we utilize scattering-based scanning near-field optical microscopy (s-SNOM) [24] to visualize and investigate mid-IR phonon polaritons in BNNTs ( Fig. 1d and Methods). s-SNOM has been previously used to study phonons [25] and SPhPs in planar materials [19] , [26] , [27] . In this technique, a sharp metallic probe produces an optical near-field with high spatial frequencies that enables sub-diffraction limit imaging with 10 nm spatial resolution. The apparatus is capable of simultaneously imaging the topography with atomic force microscopy (AFM), a capability that is used to obtain the shape and dimensions of chemically synthesized BNNTs deposited on a flat gold surface. As Fig. 2a illustrates, the BNNT under study is supported by another underlying BNNT. The BNNT of interest has a 25-nm diameter (profile analysis is shown in Supplementary Fig. 2 . The height of the BNNT is used to indicate the diameter; the lateral dimension from the topography image is convolved with the radius of the tip, ~10 nm). We utilize the phase-controlled homodyne technique to obtain the near-field signal that is proportional to the imaginary part of the near-field scattering signal with the choice of homodyne phase π /2 (ref. 28 ). 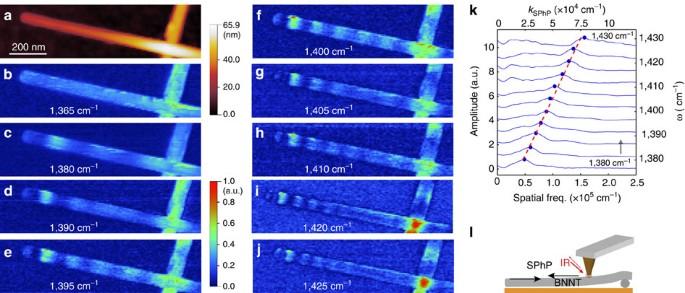Figure 2: Observation of surface phonon polariton of boron nitride nanotube. (a) AFM topography of a terminal of a BNNT on a flat gold substrate. The BNNT is supported by another BNNT in the middle. (b–j) Near-field images taken atπ/2 phase homodyne condition at 1,365, 1,380, 1,390, 1,395, 1,400, 1,405, 1,410, 1,420 and 1,425 cm−1. Nodal patterns emerge at high frequency and their separation decreases with increasing frequency, indicating a compression of the SPhP wavelength. (k) Fourier transform of the profile along the BNNT. The peak position of the spatial frequency is marked by blue dots. An increase of spatial frequencies is observed with the increase of IR frequencies. The Fourier transforms from 1,380 to 1,430 cm−1with a 5 cm−1increment offset for clarity and shown with the bottom and left axis. Corresponding dispersion relation of the BNNT SPhP is shown with top and right axis. It is constructed by correlating the spatial frequency peaks on Fourier transforms with laser excitation wavelengths considering the nodal pattern generation scheme shown inl. A numeric simulated dispersion relation of SPhP is plotted as the red dashed curve ink; the effective tube-substrate separation is assumed to be 2.5 nm. Figure 2: Observation of surface phonon polariton of boron nitride nanotube. ( a ) AFM topography of a terminal of a BNNT on a flat gold substrate. The BNNT is supported by another BNNT in the middle. ( b – j ) Near-field images taken at π /2 phase homodyne condition at 1,365, 1,380, 1,390, 1,395, 1,400, 1,405, 1,410, 1,420 and 1,425 cm −1 . Nodal patterns emerge at high frequency and their separation decreases with increasing frequency, indicating a compression of the SPhP wavelength. ( k ) Fourier transform of the profile along the BNNT. The peak position of the spatial frequency is marked by blue dots. An increase of spatial frequencies is observed with the increase of IR frequencies. The Fourier transforms from 1,380 to 1,430 cm −1 with a 5 cm −1 increment offset for clarity and shown with the bottom and left axis. Corresponding dispersion relation of the BNNT SPhP is shown with top and right axis. It is constructed by correlating the spatial frequency peaks on Fourier transforms with laser excitation wavelengths considering the nodal pattern generation scheme shown in l . A numeric simulated dispersion relation of SPhP is plotted as the red dashed curve in k ; the effective tube-substrate separation is assumed to be 2.5 nm. Full size image In the absence of phonon polaritons, the imaginary part of the near-field response relates to the light extinction that is associated with the local IR absorbance. At the IR frequency of 1,365 cm −1 , the near-field image ( Fig. 2b ) shows spatially homogeneous BN absorption (see Supplementary Fig. 3 for the Fourier transform infrared spectrum). On the high frequency side of the BN phonon resonance, the phonon polaritons emerge. The metallic AFM tip locally enhances the IR field and provides high-momentum components to launch SPhPs that propagate along the BNNT. On reaching the tube terminal, the SPhPs are reflected back toward the AFM tip and interfere with the incident polaritons, creating a standing-wave pattern depending on the position of the AFM tip relative to the BNNT terminal. Such a mechanism is conceptually similar to related near-field observations of graphene plasmons [12] , except the nanotube is a one-dimensional material. A series of near-field images of the nanotube collected at IR frequencies ω ranging from 1,380 to 1,425 cm −1 are shown in Fig. 2c–j , exhibiting alternating crests (peaks) and nodes (valleys). The separation between two consecutive nodes (peaks) corresponds to half a polariton wavelength λ ph . At 1,380 cm −1 , the phonon polaritons have a comparatively long wavelength of 400 nm. The nodal pattern progressively compresses at higher IR frequencies, suggesting that the polariton wavelength shrinks with increasing excitation frequency. For instance, λ ph is ~325 nm at 1,385 cm −1 , and decreases to λ ph ~143 nm at 1,425 cm −1 . The Fourier transforms ( Fig. 2k ) of the near-field profiles clearly demonstrate the blue-shift of the nodal spatial frequency with increasing IR excitation frequencies. Simultaneously, a decrease of polariton propagation distance is discernable from the near-field images. Between 1,380 and 1,400 cm −1 , nodal patterns are observed between the terminal and the point where the BNNT is supported by the underlying tube. At 1,405 and 1,410 cm −1 , the nodal pattern barely reaches the underlying tube. At higher frequencies of 1,420 and 1,425 cm −1 , the nodal pattern only extends to about half of the distance between the terminal and the underlying tube. These observations suggest that polaritons with shorter wavelengths experience higher attenuation. The dispersion relation of the BNNT phonon polariton is experimentally obtained by correlating 1/ λ ph with the excitation frequency ω ( Fig. 2k ). The group velocity of the SPhPs is estimated to be 3.0 × 10 5 m s −1 , about 0.1% of the speed of light in vacuum. Such a group velocity stems from strong lattice activity at mid-IR frequencies which may underlie the exceptional thermal conductivity of BNNTs [29] , [30] . The effective index (field confinement factor) is defined by n eff = λ 0 / λ ph , where λ 0 is the free space wavelength. The near-field images indicate that n eff varies from n eff =18 at 1,380 cm −1 to n eff =49 at 1,425 cm −1 . The field confinement factor is found to be higher than that is achieved by two-dimensional h -BN [19] , while the attenuation is also higher. SPhPs from multiple BNNTs of different diameters on a gold substrate have been measured (for example, Supplementary Figs 4 and 5 ). At a fixed IR frequency, a trend of increasing effective index with decreasing tube diameter D is found ( Fig. 3a )—very large effective index values are measured, up to n eff ~70. As a result, nanometre-size tubes help achieve higher field confinement than simple planar materials, which is analogous to nanofocusing in plasmonics. [9] Other phonon polariton materials, for example, SiC, if produced in the 1D nanotube form, should also provide a high effective index ( Supplementary Fig. 6 ). 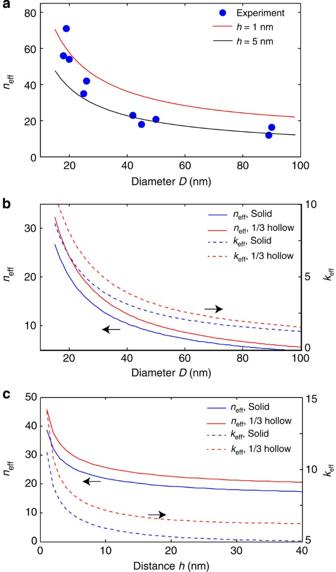Figure 3: Tailoring of surface phonon polariton property. (a) Experimentally extracted BNNT diameterDversus effective indicesneffat 1,410 cm−1on gold substrates, plotted with two simulation curves as upper and lower guides with different diameter and tube-substrate separation h. Tubes in the simulations are assumed to be 1/3 hollow. Small diameter tubes are more likely to conform to the substrate, and therefore have smaller tube-substrate separations. (b) Variation of the SPhPs complex effective index for solid and 1/3 hollow BNNTs in air as a function of the BNNT diameterD. (c) Variation of the SPhPs complex effective index of 25 nm diameter solid and 1/3 hollow BNNTs as a function of the BNNT distance h to a flat gold substrate. Figure 3: Tailoring of surface phonon polariton property. ( a ) Experimentally extracted BNNT diameter D versus effective indices n eff at 1,410 cm −1 on gold substrates, plotted with two simulation curves as upper and lower guides with different diameter and tube-substrate separation h. Tubes in the simulations are assumed to be 1/3 hollow. Small diameter tubes are more likely to conform to the substrate, and therefore have smaller tube-substrate separations. ( b ) Variation of the SPhPs complex effective index for solid and 1/3 hollow BNNTs in air as a function of the BNNT diameter D . ( c ) Variation of the SPhPs complex effective index of 25 nm diameter solid and 1/3 hollow BNNTs as a function of the BNNT distance h to a flat gold substrate. Full size image Numerical analysis of SPhPs in BNNTs To elaborate on the nature and predict the characteristics of the SPhPs, numerical analysis is conducted using the finite element method to determine the electromagnetic properties of BNNTs. The simulations in Fig. 3b shows that for an isolated tube, the mode’s effective index rapidly increases for smaller BNNTs, at a cost of higher propagation loss. Furthermore, hollowed BNNTs produce more confined modes due to further field penetration into the hollow core. As a property of multiwall nanotubes, tube hollowness allows the fine-tuning of SPhP properties, while maintaining external geometries of the tube (transmission electron microscopy images of BNNTs of the same batch shown in Supplementary Fig. 7 provide the estimation of the size of hollow cores for numerical simulations). While the mode of a suspended BNNT possesses azimuthal symmetry, introduction of a substrate breaks the symmetry and squeezes the mode between the BNNT and the substrate as shown in the right-hand panels of Fig. 1d . This behaviour translates to even higher effective indices and is more pronounced for a conductive substrate like gold. Figure 3c quantifies this effect and also explains the large experimentally observed n eff of Fig. 3a . The loss k eff also generally increases with field confinement, a trade-off that is consistent with (and well-known in) plasmonics. Corresponding numerical simulations on the field enhancement of BNNT as a function of tube diameter and tube-substrate separation are included in Supplementary Fig. 8 . The dispersion of the SPhPs as a function of the excitation frequency was also computed and is plotted in Fig. 2k (red dashed), showing an increase in n eff with an increase in IR frequency. Strong dispersion is normally accompanied by strong dissipation, as can be understood from the Kramers–Kronig relation between the real and imaginary parts of the dielectric function, explaining the observed change in the attenuation over this frequency range. Compensation of SPhP loss with a rough metallic surface The dielectric property and local geometry of the substrate affect the generation and propagation of SPhPs in BNNTs ( Supplementary Figs 9–11 and Supplementary Note 2 ). 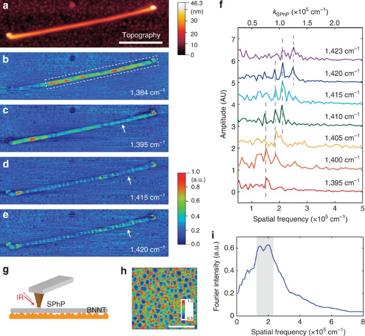Figure 4: SPhPs of a BNNT on a rough gold surface. (a) AFM topography of a BNNT of 19 nm diameter on a rough gold substrate. (b–e) Near-field images are obtained with IR frequencies 1,384, 1,395, 1,415 and 1,420 cm−1. The scale bar is 500 nm. Nodal separation (marked by the white arrow) decreases with increasing laser frequencies. The periodical nodal patterns extend along the whole tube at 1,420 cm−1, rather than showing decays in the short range inFig. 2i. (f) Fourier transforms of the nodal patterns of multiple IR frequencies from the tube segment marked by the white dashed box in (b). UnlikeFig. 2k, the Fourier transform reveals multiple spatial frequencies. This is due to multiple SPhP launching sites. (g) Scheme of a BNNT on rough gold surface. (h) Near-field image of the rough gold substrate. The scale bar is 200 nm. (i) Radially averaged two-dimensional Fourier transform ofh, showing a distribution of spatial frequencies. The range of spatial frequencies of the SPhP is marked by the grey box. The analysis of the substrate roughness and phenomenological signal generation mechanism are described inSupplementary Fig. 12andSupplementary Note 3. Figure 4a–e shows topography and near-field images taken at frequencies 1,384, 1,395, 1,415 and 1,420 cm −1 of a BNNT of 19 nm diameter on a rough gold surface. Nodal patterns characteristic of SPhPs are observed. The spatial frequencies of nodal patterns increase with increasing IR frequencies. Corresponding spatial frequencies are obtained through Fourier transforms ( Fig. 4f ). The thin tube diameter again leads to high effective indices, as high as 60 at 1,395 cm −1 and 77 at 1,420 cm −1 . However, the standing-wave patterns of BNNT SPhPs, herein, extend over a much longer distance compared to those on the smooth gold surface. For example, at a frequency of 1,420 cm −1 , the SPhP associated with the 25 nm diameter BNNT on the smooth gold exhibited a decay length of~300 nm ( Fig. 2i ), whereas the 19 nm diameter BNNT on the rough gold substrate supports a nodal patterns spanning the entire 1.9 μm length of the nanotube. The spectral content of these long-range nodal patterns consists of a set of sharp Fourier peaks ( Fig. 4f ), in contrast to a single broad spatial frequency peak for BNNTs on the smooth gold substrate ( Fig. 2k ). In addition, the position of these sharp peaks in the momentum space is virtually fixed for adjacent IR excitation frequencies—(marked by the vertical dashed lines in Fig. 4f ). These spectral features and the increased extent of the SPhP standing waves are profoundly correlated. Figure 4: SPhPs of a BNNT on a rough gold surface. ( a ) AFM topography of a BNNT of 19 nm diameter on a rough gold substrate. ( b – e ) Near-field images are obtained with IR frequencies 1,384, 1,395, 1,415 and 1,420 cm −1 . The scale bar is 500 nm. Nodal separation (marked by the white arrow) decreases with increasing laser frequencies. The periodical nodal patterns extend along the whole tube at 1,420 cm −1 , rather than showing decays in the short range in Fig. 2i . ( f ) Fourier transforms of the nodal patterns of multiple IR frequencies from the tube segment marked by the white dashed box in ( b ). Unlike Fig. 2k , the Fourier transform reveals multiple spatial frequencies. This is due to multiple SPhP launching sites. ( g ) Scheme of a BNNT on rough gold surface. ( h ) Near-field image of the rough gold substrate. The scale bar is 200 nm. ( i ) Radially averaged two-dimensional Fourier transform of h , showing a distribution of spatial frequencies. The range of spatial frequencies of the SPhP is marked by the grey box. The analysis of the substrate roughness and phenomenological signal generation mechanism are described in Supplementary Fig. 12 and Supplementary Note 3 . Full size image As Fig. 4h illustrates, the rough gold surface consists of randomly placed densely packed nanometre-sized grains of diameters ranging from 10 to 30 nm. The roughness, in turn, can provide the momentum required for the excitation of SPhPs along the BNNTs, a mechanism unavailable to BNNTs on a smooth gold substrate. The sharp Fourier peaks associated with the SPhP standing waves ( Fig. 4f ) clearly fall within the spectral bandwidth of the substrate roughness ( Fig. 4i ), centred at G ≈1.8 × 10 5 cm −1 . Moreover, it can be readily seen that these sharp peaks correspond to wavenumbers, G , nearly satisfying the Bragg condition G ≈2 k SPhP Therefore, it is apparent that the observed long-range standing-wave SPhP patterns are due to the constructive interference of roughness-mediated excitations along the BNNTs at multiple points. The model of constructive interference with Bragg condition is consistent with the observed linear power dependence of SPhP intensity verses input laser power ( Supplementary Fig. 13 ). On the other hand, those components resulting in destructive interference are severely suppressed. This explains the substantial extension of the SPhPs standing-wave patterns along the BNNTs as well as their sharper spectral content and milder dispersion compared to those of the smooth-substrate SPhPs. Coupling through roughness is of practical interest because it is easy to achieve, and because it allows incident light to be coupled to the nanotube over its entire length, compensating effectively the propagation loss. The presence of SPhPs in BNNTs contributes the nanoscopic IR spectra at the SPhP frequencies (see Supplementary Fig. 14 and Supplementary Note 4 ). BNNT structural variations cause more obvious spectral variations at SPhP frequencies than at the BN phonon frequencies [28] . In particular, a local structural defect of a BNNT scatters SPhPs, leading to enhanced near-field absorption at the site of the defect at the SPhP frequencies (marked by the white circle in Supplementary Fig. 14c ). Detection of SPhPs could be used to identify local structural defects of BNNT to monitor fabrication quality for quality control purpose. In summary, we have demonstrated excitation and propagation of 1D mid-IR SPhP in BNNTs by means of s-SNOM. It has been experimentally and theoretically shown that the SPhPs possess short polariton wavelengths and very large effective indices, they are highly confined and provide substantial field enhancement, all of which are very desirable for a variety of applications including near-field imaging, sensing, nonlinear optics, surface spectroscopy, and nano-optics. The modal characteristics of the BNNT SPhPs may be controlled through their geometrical and structural attributes, the choice of substrate, as well as the separation from the substrate. The loss can be mitigated with the use of a rough gold substrate or possibly a periodic substrate, by coupling light over the length of the tube. These findings show the potential of BNNTs as a viable means for utilizing 1D SPhPs. IR near-field nanoimaging apparatus The layout of the apparatus is shown in Supplementary Fig. 15 . A quantum cascade laser (Daylight Solutions) is used to provide a continuous wave, frequency tunable optical signal of 50 mW at mid-IR frequencies. The laser frequency is tuned to the high frequency side of the BN phonon resonance of 1,363 cm −1 (see Supplementary Fig. 1 for the Fourier transform infrared spectrum). An atomic force microscope (Multimode AFM, Bruker Nano) is modified to allow for optical access to its probe tip. A metal-coated tip (DPE-14 Mikromash) is used to enhance the light field at its apex through near-field localization. The AFM operates in tapping mode with the tip oscillating vertically above the sample at Ω=156 kHz with an amplitude of 30 nm. The mid-IR laser light is focused to and collected from the tip and sample region using a parabolic mirror with effective numeric aperture of 0.24. The collimated scattered light is interferometrically homodyned with a reference laser field from the same source. An IR detector (J15D12, Teledyne-Judson) is used to convert the optical field into an electric signal that is demodulated by a lock-in amplifier (HF2Li Zurich instrument) at the third harmonic of the vertical oscillation frequency (3Ω) of the tip. The π /2 homodyne phase condition is set by minimizing the near-field signal from the gold substrate, as described previously [28] . A phase feedback device is used to stabilize the homodyning phase. The choice of the homodyne phase does not affect the read-out of nodal periodicities of BNNT SPhPs ( Supplementary Fig. 16 and Supplementary Note 5 ). The spatial resolution of the near-field apparatus is found to be about 10 nm ( Supplementary Fig. 17 ). Numerical analysis and electromagnetic modelling COMSOL Multiphysics is used for the numerical analysis and electromagnetic modelling of the BNNTs based on the finite element method. Sub-nanometre mesh sizes are used to discretize the BNNT and its immediate vicinity, including the air hole of hollow nanotubes. Variation of the eigenvalues as a function of the mesh size is monitored to ensure convergence of the results. The dielectric functions for Au and SiO 2 , SiC and BN are, respectively, taken from Palik [31] , Le Gall et al. [23] , and Geick et al. [18] Sample synthesis and preparation The multiwall BNNTs are synthesized by using a high-temperature chemical vapour deposition synthesis in an induction furnace. More details may be found in the literature [32] . In brief, MgO, SnO (or FeO) and B powders at a weight ratio of 7:150:30 were thoroughly mixed, placed in a BN crucible and heated by the induction currents up to 1,400–1,500 °C in flow of Ar carrying gas and NH 3 reactive gas. The obtained snow-white BN product is purified by annealing in an Ar atmosphere at 1,900 °C in an induction furnace. The BNNTs are dispersed in isopropanol with sonication for 5 h and drop casted on a flat gold substrate (rms. roughness 1.7 nm over a 100 nm by 600 nm area), and a rough gold substrate (SSENS Bv). How to cite this article: Xu, X. G. et al. One-dimensional surface phonon polaritons in boron nitride nanotubes. Nat. Commun. 5:4782 doi: 10.1038/ncomms5782 (2014).